Variability in the quality of visual working memory Working memory is a mental storage system that keeps task-relevant information accessible for a brief span of time, and it is strikingly limited. Its limits differ substantially across people but are assumed to be fixed for a given person. Here we show that there is substantial variability in the quality of working memory representations within an individual. This variability can be explained neither by fluctuations in attention or arousal over time, nor by uneven distribution of a limited mental commodity. Variability of this sort is inconsistent with the assumptions of the standard cognitive models of working memory capacity, including both slot- and resource-based models, and so we propose a new framework for understanding the limitations of working memory: a stochastic process of degradation that plays out independently across memories. Working memory is critical to navigation, communication, problem solving and other activities but there are stark limits to how much we can remember [1] , [2] , [3] , [4] , [5] , [6] , [7] , [8] , [9] . A goal of research on working memory is to describe these limitations and determine their source. Cognitive models typically explain the capacity of working memory by postulating a mental commodity that is divided among the items or events to be remembered [1] , [3] , [5] , [9] , [10] , [11] , [12] . A core assumption of these models is that the quality (‘fidelity’, ‘uncertainty’) of memories is determined solely by the amount of the commodity that is allocated to each item, being otherwise fixed [1] , [5] , [10] , [11] , [12] , [13] . Items receiving more of the commodity are better remembered. A common approach to measuring the capacity of visual working memory is through the use of simple behavioral tasks. In one such task, participants are asked to remember the colours of a set of colourful dots, and then, after some delay, to report the colour of a dot selected at random ( Fig. 1 ) [1] , [9] . Error is recorded as the difference between the correct colour and the reported colour. The distribution of these errors is used to test models of memory. Standard models [1] , [5] , [10] , [11] , [12] , [13] assume that for each dot in the display, the participant is in one of two states, either remembering or forgetting. Importantly, these two states lead to different errors when the participant is asked to report the dot’s colour: errors for a forgotten item are uniformly distributed on the colour wheel, whereas errors for a remembered item cluster around the correct colour, with a spread that depends on how well it was remembered. The standard models assume that the form of the error distribution for remembered items is a circular normal (von Mises) distribution, with a spread that can be fully characterized by a single number: its precision, here defined as the s.d. (ref. 1 ). 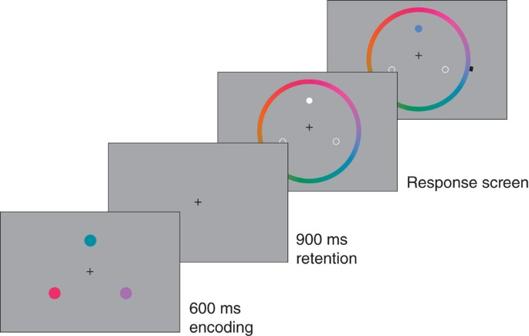Figure 1: Timeline of a working memory task. First, a display of colourful dots is briefly presented (lower left). This is followed by an interval during which the participant is asked to hold the colours in mind. Finally, a response screen appears. On the response screen, the position of a randomly sampled item is cued and the participant is asked to select the colour of the item that was presented at that location (upper right). Figure 1: Timeline of a working memory task. First, a display of colourful dots is briefly presented (lower left). This is followed by an interval during which the participant is asked to hold the colours in mind. Finally, a response screen appears. On the response screen, the position of a randomly sampled item is cued and the participant is asked to select the colour of the item that was presented at that location (upper right). Full size image It is possible to relax the assumption that the quality of memory is fixed, instead supposing that it varies within an individual. To determine whether such variability is present, we can inspect the shape of the error distribution. Critically, variability in the precision of memory within an individual leads to an error distribution that is more peaked than a circular normal distribution because it involves mixing error distributions that differ in precision but have the same mean ( Fig. 2 ). With sufficient data, it is possible to measure this peakedness to estimate the extent of high-order variability in the quality of memory within an individual. 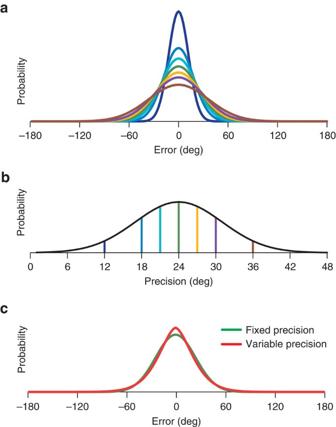Figure 2: Fixed and variable-precision models produce different distributions of error. (a) Each curve shows the distribution of precision (the s.d. of error on the memory task) for a different fixed-precision model. (b) A variable-precision model can be thought of as a higher-order distribution of fixed-precision models. One such higher-order distribution is shown here; it is a truncated normal with a mean of 24° and a s.d. of 7°, bounded at 0° and 100°. (c) Variable-precision models have different distributions of error. The green line is the distribution of errors for a model whose precision is fixed at 24°. (The green distribution in panelsaandcare the same.) The red line is the expected distribution of errors if precision were drawn from the full distribution in panelb. Mixing together distributions with different precision produces a peaked shape that is a hallmark of the variable-precision model. Figure 2: Fixed and variable-precision models produce different distributions of error. ( a ) Each curve shows the distribution of precision (the s.d. of error on the memory task) for a different fixed-precision model. ( b ) A variable-precision model can be thought of as a higher-order distribution of fixed-precision models. One such higher-order distribution is shown here; it is a truncated normal with a mean of 24° and a s.d. of 7°, bounded at 0° and 100°. ( c ) Variable-precision models have different distributions of error. The green line is the distribution of errors for a model whose precision is fixed at 24°. (The green distribution in panels a and c are the same.) The red line is the expected distribution of errors if precision were drawn from the full distribution in panel b . Mixing together distributions with different precision produces a peaked shape that is a hallmark of the variable-precision model. Full size image Here, using variants of the behavioral task outlined, in Figure 1 we show that there is variability in the quality of working memory within an individual. This variability can be explained neither by fluctuations in attention or arousal over time, nor by uneven distribution of a limited mental commodity. We propose that a complete understanding of the capacity and architecture of working memory must consider both the allocation of a mental commodity and the stability of the information that is stored. Revealing variability in the quality of working memory Participants were asked to perform a working memory task using displays with 1, 3 or 5 colourful dots ( Fig. 1 ). The standard fixed-precision model [1] and our variable-precision model was fit to each participant’s distribution of errors (see Methods). 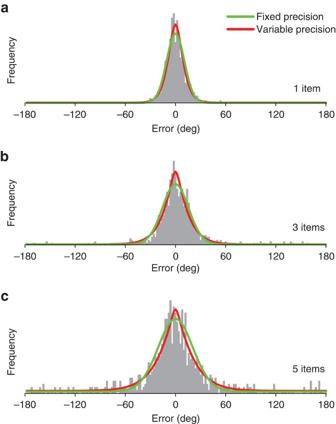Figure 3: Distinguishing between models with fixed and variable precision. Each panel shows a histogram of errors on the working memory task and the best-fit fixed precision (green line) and variable-precision (red line) model. The working memory task used 1, 3 or 5 items (panelsa,bandc, respectively). These data are from a representative participant. Figure 3 overlays the maximum a posteriori fixed- and variable-precision models on a histogram of errors made by one of the participants, for each of three set sizes: 1, 3 and 5. The variable-precision model provided a better fit to the data for each participant at each set size. When the two models were compared using the Akaike Information Criterion (AIC), a measure of goodness of fit, we found lower AIC values for the variable-precision model for each participant at each set size ( Supplementary Table S1 ); the average magnitude of these AIC differences (7, 11.3 and 12) is a decisive victory for the variable-precision model, leaving the fixed-precision model with ‘essentially no support’ from the data [14] . Furthermore, the amount of variation in memory precision increased with set size for each participant ( Fig. 4 ). The average precision across subjects was 11.6°, 17.4° and 23.7° for set sizes 1, 3 and 5, respectively. The average s.d. of precision, a measure of variability in memory quality, was 3.0°, 5.4° and 8.9°. These results were obtained with a variable-precision model in which the variability in precision was assumed to follow a truncated normal distribution. Evidence of variable quality was also found when substituting a gamma distribution over the inverse of the variance, similar to [15] (average inverse variance 0.0091, 0.0051, 0.0031, deg −2 ; average s.d. of inverse variance, 2.3 × 10 −5 , 1.1 × 10 −5 , 9.0 × 10 −6 deg −2 ). Figure 3: Distinguishing between models with fixed and variable precision. Each panel shows a histogram of errors on the working memory task and the best-fit fixed precision (green line) and variable-precision (red line) model. The working memory task used 1, 3 or 5 items (panels a , b and c , respectively). These data are from a representative participant. 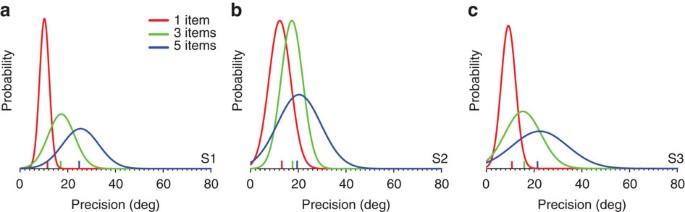Figure 4: Variability in the quality of working memory depends on the load. The estimated distribution of precision according to the best-fitting variable-precision model for set sizes 1 (red), 3 (green) and 5 (blue), for each of three subjects (panelsa–c). The bars along the horizontal axis show the precision values of the best-fit fixed-precision models. Full size image Figure 4: Variability in the quality of working memory depends on the load. The estimated distribution of precision according to the best-fitting variable-precision model for set sizes 1 (red), 3 (green) and 5 (blue), for each of three subjects (panels a – c ). The bars along the horizontal axis show the precision values of the best-fit fixed-precision models. Full size image Determining the source of the variability There are many possible sources of variability, including both true variability in memory precision as well as variability from other sources, such as perceptual noise, eye movements and differences in the memorability of certain colours or locations. A series of control experiments were performed that demonstrate that these other sources made only a negligible contribution to the observed variability in memory quality. When the memory demands of the task were removed by keeping the stimulus present while the participant responded, variability was eliminated and the data were better fit by a fixed-precision model ( Supplementary Table S2 ). Even when the average error on the perception task was increased to match that of the memory task ( Supplementary Methods ), variability was still smaller (2.2° versus 8.9°, t (4)=3.86, P <0.05, independent samples t -test). A further experiment showed that there were negligible differences in the memorability of different colours ( Supplementary Methods ). We measured the variation in precision for six colour bins, each spanning 30° of the colour wheel (0–30°, 60–90°, …, 300–330°). Even though the range of colours within each bin was now only a small subset of the colour wheel, we still found substantial variability within a bin ( Supplementary Fig. S1 ). In fact, the variability within a bin was comparable to that in the full data set ( Supplementary Fig. S1c , one-sample t -tests, all t (5)’s <0.5, all P >0.65 for both participants). Furthermore, the variation in estimates of precision across bins was minimal and accounts for at most a small (3.9%) portion of the total variance. Similarly, we tested whether performance differed depending on the location of the tested item, a possible contributor to the observed variability in memory. For both the three- and five-item displays, we found little variance in the estimated precision across locations (4.15 deg 2 for three-item displays, 3.24 deg 2 for five-item displays). (This is an upper bound on the contribution to variance because it includes measurement error.) Furthermore, the observed variance explains only 12.7% and 3.8% of the total variance for the three-item and five-item conditions, respectively. Representational quality could differ for items that are fixated compared with items that are not. The encoding duration used in Experiment 1 was long enough to allow for a saccade, therefore raising the possibility that variability in precision is due entirely to imbalances in encoding introduced by eye movements. We found that memories are variably precise even when eye movements are not possible. Two participants were asked to remember the colour of three items presented for 100 ms. Although this encoding duration is too short for an eye movement, we nonetheless found variability in the precision of working memory. Both participants’ data were better fit by the variable- than fixed-precision model (average difference in AIC c values of 4.0 in favour of the variable-precision model). The previous manipulation eliminated the possibility of eye movements during stimulus presentation, but it does not address the possibility that gaze was not centered on fixation. We performed an additional follow-up experiment in which stimulus presentation was conditional on 1,000 ms of continuous, uninterrupted fixation ( Supplementary Methods ). The data for two out of the three participants were better fit by the variable- than fixed-precision model, with an average difference in AIC c of 6.7 in favour of the variable-precision model. There is variability between items within a trial In the following experiments, we show that this variability can be explained neither by state-based fluctuations in attention or arousal across trials [16] , nor by the uneven allocation of a mental commodity within a trial. This pattern of results is not easily captured by models of working memory in which the quality of a memory is determined solely by the allocation of a finite commodity. In a new experiment, on half of the trials participants were given the opportunity to report the colour of the item they remembered best. On the other half of the trials, they reported the colour of an item that was selected for them at random. These two conditions were intermixed in random order. Note that only variability within a trial can contribute to the participant’s decision in this task. Therefore, if this variability is accessible to the participant, precision will be better for the best-remembered item than for one selected at random. This enables us to measure the extent to which the quality of memory varies within versus across trials. When probed on a random item, the mean precision was 19.9±1.2° (s.e.m.) and its s.d. was 6.2±0.60° ( Fig. 5a ). However, when given the opportunity to choose which item to report, the mean precision was better (15.4±0.75°, paired samples t -test, t (9)=5.3, P <0.001) and less variable (4.4±0.38°, t (9)=3.4, P =0.01) ( Fig. 5b ). 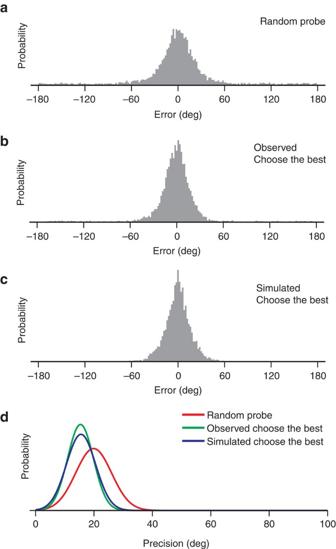Figure 5: Choosing the item that was remembered best. (a) When participants were asked to report an item selected at random, they made errors. (b) When allowed to report the item they remembered best, they performed better, seen as a narrower distribution of error. The ability to pick out the best-remembered item is evidence that the items differed in how well they were remembered. (c) Using the distribution in panela, we simulated the distribution of errors that we would expect to find in panelbif participants had perfect metamemory, always picking out the best-remembered item. (d) The observed and simulated distributions of memory quality match, suggesting that participants have nearly perfect metamemory. Figure 5: Choosing the item that was remembered best. ( a ) When participants were asked to report an item selected at random, they made errors. ( b ) When allowed to report the item they remembered best, they performed better, seen as a narrower distribution of error. The ability to pick out the best-remembered item is evidence that the items differed in how well they were remembered. ( c ) Using the distribution in panel a , we simulated the distribution of errors that we would expect to find in panel b if participants had perfect metamemory, always picking out the best-remembered item. ( d ) The observed and simulated distributions of memory quality match, suggesting that participants have nearly perfect metamemory. Full size image This outcome provides an existence proof of within-trial variability and implies that it is cognitively present and useful. But how much of the variation is contained within a trial, and how much of it is across trials? To answer this question, we ran simulations under conditions of purely within- and purely across-trial variability ( Fig. 5c ; see Methods). We did not find a difference between the observed distribution and the simulated distribution for purely within-trial variation, either in mean (15.4° observed versus 15.5±0.75° simulated; paired samples t -test , t (9)=0.05, P >0.85) or s.d. (4.4° observed versus 5.0°±0.41° simulated; t (9)=1.21, P >0.25) ( Fig. 5d ). Nor did we find a difference in the mean or s.d. of precision between the trials in which a random item was probed and trials in another control experiment, run with ten new participants, that did not include a ‘choose the best’ condition (19.9° versus 22.1±1.18°, independent samples t -tests, t (18)=0.91, P =0.38; 6.2° versus 6.0±0.74°, t (18)=0.74, P =0.48). This suggests that giving the participant the opportunity to choose the best-remembered item on some trials did not alter how items were encoded on the other trials. In showing that nearly all of the variability in memory quality is accessible to the participant on a single trial, these results rule out a sizeable contribution of across-trial variability in the present study and suggest near-perfect metamemory for the relative quality of working memory representations. These findings also speak to an alternative account of the results of the first experiment, where we found that the distribution of response error was more peaked than is predicted by standard fixed-precision models [1] , [5] , [10] , [11] , [12] , [13] . Is it possible that the distribution’s peaked shape arose not because of variability in precision, but because of a fixed-precision error distribution that is naturally more peaked than a circular normal distribution? The results of the current experiment make this alternative account unlikely because nearly all of the peakedness in the distribution of report error is accounted for by variability across items within a trial, suggesting that the peakedness of the error distribution reflects variability across items and leaving little reason to posit an additional source. Variability in memory quality is independent across items Many theories hold that the quality of a memory is determined by the allocation of a finite commodity, where items receiving more of the commodity are better remembered [1] , [3] , [5] , [9] , [12] . These theories predict that some of the within-trial variation in precision can be accounted for by uneven allocation: when more of the commodity has been allocated to one item, less is available for the others, thereby producing tradeoffs between items within a display. To determine whether the variability we observed was due to uneven commodity allocation, we performed an experiment in which participants were asked to report the colour of every item in the display. We then tested for tradeoffs by comparing the errors made for one item when the response to another item was good versus bad (that is, above versus below the median absolute error for that response across trials) ( Fig. 6 ). We found no difference in precision between above-median and below-median splits for any combination of items, regardless of whether the estimates of precision were derived from the fixed-precision model ( Fig. 7a ) (paired samples t -tests, all t (15)’s<1.6 and all P >0.1) or the variable-precision model ( Fig. 7b ) (all t (15)’s<1.2 and all P >0.25). 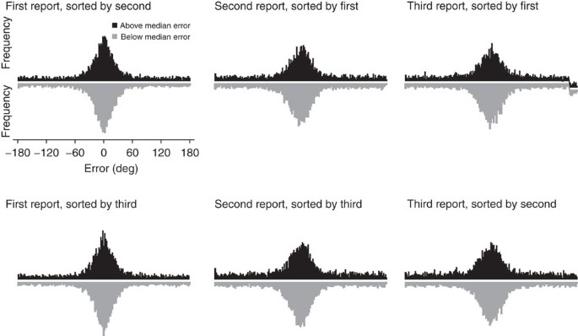Figure 6: Evidence that memory degradation is independent across items. Distributions of report error for the first, second and third responses sorted by whether the response to another item in the trial was below (black) or above (gray, flipped) the median error. Memory quality does not differ between the two, which is evidence of memory degradation that is independent across items. Figure 6: Evidence that memory degradation is independent across items. Distributions of report error for the first, second and third responses sorted by whether the response to another item in the trial was below (black) or above (gray, flipped) the median error. Memory quality does not differ between the two, which is evidence of memory degradation that is independent across items. 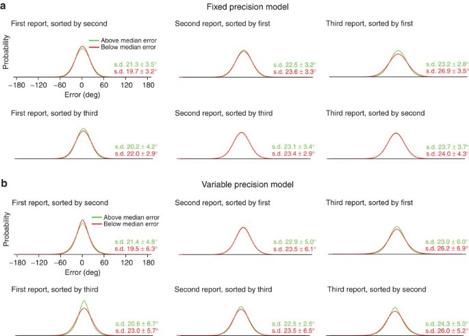Figure 7: Model fits for distributions of report error. (a)We separately fit a fixed-precision model to the data from each participant, response (first, second or third), sorting and split (above versus below the median error). The best-fit s.d. did not differ between the splits, which means that memory quality was comparable.(b)We did the same using the variable-precision model and found the same result: evidence of memory degradation that is independent across items. Full size image Figure 7: Model fits for distributions of report error. (a) We separately fit a fixed-precision model to the data from each participant, response (first, second or third), sorting and split (above versus below the median error). The best-fit s.d. did not differ between the splits, which means that memory quality was comparable. (b) We did the same using the variable-precision model and found the same result: evidence of memory degradation that is independent across items. Full size image This evidence of independence is based on a null result. However, using Monte Carlo simulations we found that our tradeoff-detection method is powerful enough to reliably detect tradeoffs if they were to exist ( Supplementary Notes and Methods ). We considered two sources of tradeoffs: (1) noiseless uneven allocation, where the participant knowingly attends or gives preferential processing to a chosen item, and (2) noisy even allocation, where the participant tries to distribute her resources evenly, but fails, unwittingly giving preference to some items over others. We found that any unevenness strong enough to produce the observed variability in precision would have been readily detected through our procedure for detecting tradeoffs ( Supplementary Notes and Methods ). Finding independence of precision for items within a display [17] , [18] rules out that the observed variability in precision reflects unevenness in the allocation of discrete slots [1] or a graded resource [5] . Visual working memory is not perfect. Its imperfections have been used to fashion cognitive models of visual working memory in which the quality of a memory is determined solely by the amount of a mental commodity that it receives. In contrast to the predictions of these models, the present results show that even under conditions of even allocation, the quality of working memory varies across trials and items. This finding is consistent with a stochastic process that degrades memory for each individual item and plays out independently across them. The outcome of this process leaves each memory in its own state, with its own precision, which when combined across items, produces the characteristic peaked shape of report-error distributions. Thus, visual working memory is stochastic both at the level of a memory’s content and at the level of its quality. A physiological mechanism that might account for variability in the quality of working memory representations is cortical noise that impedes the sustained activation of the neural populations that code for the remembered information [5] , [12] , [19] , [20] , [21] , [22] , [23] . The precision of memory representations may correspond to the amount of signal drift over time and the extent to which noisy signals are pooled within a neural population [1] , [5] , [9] , [20] , [24] , [25] , [26] . The recruitment of larger neural populations will improve the precision of working memory representations through decreased signal drift or increased redundancy in coding. Critically, the probability that neurons within a population will self-sustain after stimulus offset is known to be affected by internal noise [20] , [21] , [22] . Under these circumstances, the precision of memory representations would be determined by the outcome of stochastic physiological processes operating independently across representations. Existing models explain the source of limitations in working memory solely by reference to a finite capacity for storing information. Here, we have shown that a complete account of visual working memory must also consider the stability of stored information. To put forward one model capable of producing variability of the sort described here, consider a finite mental commodity that must be divided among the items to be remembered. As in existing models, this information limit can be formalized as a set of N independent samples that are allocated to the items being remembered [1] , [9] , [10] , [11] , [12] , with slot models setting N to ∼ 3, and with continuous resource models considering the limit as N tends to infinity. Suppose that the samples are unstable and that each has some probability of surviving until the time of the test. This leads to variability in memory quality of a specific form: a binomial distribution of samples per item. This random process, known as the pure death process in studies of population genetics, is one of many possible random processes that might degrade memory. Our model includes a guess state, a catch-all for trials in which the participant guesses randomly, either because of lapses in memory or because of other hiccups, such as blinks and slips of the hand. A recent paper [15] has suggested that allowing for variability in the quality of working memory obviates the need to include a guess state. Though we agree that there is risk of overestimating the rate of guessing if variability is ignored, we found that even taking variability into account, a guess state still accounts for a sizeable proportion of trials ( Supplementary Notes and Methods ). Moreover, the goal of the present work is not to argue that participants never guess, but to show that variability in the quality of working memory reflects a random process of degradation that plays out independently across memories. Models of working memory that are constrained by the known properties of the brain uniformly propose that the maintenance of working memory representations involves stochastic processes that operate at all levels of processing [21] , [27] , [28] . Yet most cognitive models explain working memory solely by reference to the division of a mental commodity: a resource divided among stored items [1] , [3] , [4] , [5] , [9] , [10] , [12] . In these models, the quality of a memory representation is deterministic and based solely on the amount of the commodity allocated to it. Demonstrating independent, stochastic variation in memory quality within an individual requires a new framework that includes a role for stochastic processes, helping to bridge the gap between biologically plausible neural models on the one hand and cognitive models on the other. Participants Participants were between the ages of 18 and 28 years, had normal or corrected-to-normal vision and received either $10 per hour or course credit. Participants whose testing ran over multiple days were given a bonus of $10 per session after the first. The studies were performed in accordance with Harvard University regulations and approved by the Committee on the Use of Human Subjects in Research under the Institutional Review Board for the Faculty of Arts and Sciences. Stimuli The stimulus was 1, 3 or 5 colourful dots arranged in a ring around a central fixation mark. The radius of each dot was 0.4° in visual angle and the radius of the ring was 3.8°. Each dot was randomly assigned one of 180 equally spaced equiluminant colours drawn from a circle (radius 59°) in the CIE L * a * b * colour space, centered at L =54, a =18 and b =−8. The grouping strength of the colours was controlled by transforming the colour values to vectors in polar space, selecting displays with the constraint that the magnitude of the mean vector of each display was equal to that expected of a randomly sampled display. Presentation Stimuli were rendered by a computer running MATLAB with the Psychophysics Toolbox [29] , [30] . The display’s resolution was 1,920 × 1,200 at 60 Hz, with a pixel density of 38 pixels per cm. The viewing distance was 60 cm. The background was gray, with a luminance of 45.4 cd m −2 . Procedure On each trial, the stimulus was presented for 600 ms and then removed. After a 900-ms delay, a filled white circle appeared at the location of a randomly selected item and hollow circles appeared at the location of the other items. Participants were asked to report the probed item’s colour by selecting it from a response screen with the full colour wheel, 6.5° in radius, centered around fixation. A black indicator line was placed at the outer edge of the response wheel at the position closest to the cursor. Once the participants moved the mouse, the filled circle’s colour was continuously updated to match the currently selected colour. Participants registered their choice by clicking a mouse. Responses were not speeded. Feedback was provided after each response by displaying onscreen the error in degrees. Experiment 1 methods Three participants performed three sessions, each lasting 1.5–2 h. Each session used 1, 3 or 5 items, and their order (and therefore, set size) was counterbalanced across participants. There were 800 trials per session for set sizes 1 and 3 and 720 trials per session for set size 5. Experiment 2 methods Ten participants performed two 700-trial sessions with a set size of 3. On half of the trials, participants reported the item they remembered best. On the other half, participants reported the colour of a randomly selected item. Probe types were intermixed in random order. On ‘choose the best’ trials, instructions appeared at the top of the screen telling participants to report a colour and then to select the location of the best-remembered item by clicking its location. On these trials, filled white circles appeared at the locations of the probed and non-probed items. Experiment 3 methods A total of 16 participants performed one 500-trial session with a set size of 3. Instead of reporting only one item, participants were asked to report all three. Items were probed in random order. Feedback was given. Non-probed items, even those already reported, were indicated by hollow circles. General framework for modeling the error distribution All of the models considered here can be seen as special cases of an infinite scale mixture, a general framework that describes error distributions with a fixed mean and a precision (scale) that is sampled from some higher-order distribution, known as the ‘mixing distribution’. Fixed-precision model In the fixed-precision model, the participant is in one of two states for each item on the display. With probability 1– g , she remembers the item and has some fixed amount of information about it. Limited memory leads to errors in recall, which are assumed to be distributed according to a von Mises distribution (the circular analogue of a normal distribution) centered at zero (or, perhaps, with some bias μ ) and with spread determined by a concentration parameter κ that reflects the memory’s precision. The mixing distribution is thus the Dirac delta function at κ , a distribution concentrated at that one point. With probability g , she remembers nothing about the item and guesses randomly, producing errors distributed according to a circular uniform. Together, the probability density function of this model is given by where φ is the von Mises density, defined by where I 0 is the modified Bessel function of order zero. Variable-precision model The variable-precision model is the same as the fixed-precision model, except that precision is distributed according to some higher-order distribution, for example, a truncated normal or gamma distribution. Unless guided by a theory for the source of variability in precision, the choice of mixing distribution is arbitrary, but certain combinations of error distribution and mixing distribution are convenient. For example, when error is normally distributed about the correct value, and when precision (that is, the inverse of variance) is gamma distributed, the resulting experimental data takes the form of a generalized Student’s t -distribution. (This result generalizes to the case of distributions wrapped on the circle, which is useful for representing colours and orientations.) For guess rate g , bias μ and s.d. σ , the probability density function of this model is given by where ψ is the wrapped generalized Student’s t -distribution [31] and is given by Incorporating higher-order variability into new models of working memory is therefore a simple matter of replacing the usual choice of error distribution, a von Mises distribution, with a wrapped generalized Student’s t -distribution. Some combinations of error and mixing distributions give rise to named distributions with known analytic expressions [32] , [33] , but others, like the truncated normal mixing distribution, must be simulated. The mean precision and its s.d. were free parameters, bounded between 0° and 100°. (The upper bound is arbitrary, but an s.d. above 100° is typically indistinguishable from guesses anyways). This should not be taken as a strong claim about the form of the distribution of memory precision, which will depend crucially on the process that degrades memories. However, no matter which distribution is chosen, the presence of variability produces a signature effect on the data—peakedness in the error distribution—seen most clearly in Fig. 2 , and which is readily detected using the present methods. Model fitting Markov Chain Monte Carlo was used to find the maximum a posteriori parameter set of a model given the errors on the memory task. Each model was fit separately for each subject and experimental condition. The data were not binned. We used the Metropolis–Hastings algorithm, which takes a random walk over the parameter space, sampling locations in proportion to how well they describe the data and match prior beliefs. A non-informative Jeffreys prior was placed over each parameter. The proposal distribution used to recommend jumps was a multivariate Gaussian centered at the current parameter set, whose s.d. was tuned during a burn-in period that ended when all of the chains, which started at different locations in the parameter space, converged. We collected 15,000 samples from these converged chains and report the sample with the maximum posterior probability. Model comparison To compare the relative goodness of fit of the fixed- and variable-precision models, we computed each model’s AIC, a measure that includes a penalty term for the number of free parameters [34] . For a model with k parameters and maximum log-likelihood L , the AIC is given by Because this formulation of the AIC assumes infinite data, it is necessary to correct the value when estimating it from experimental data. The corrected AIC, AIC c , is given by where n is the sample size—that is, the number of trials performed by a participant on the working memory task. Simulating across- and within-trial variation in Experiment 2 We performed Monte Carlo simulations to estimate the distribution of precision when ‘choosing the best’ under conditions of purely across-trial variation or purely within-trial variation. For each subject, 1,000 trials (of three-item displays) were simulated according to that participant’s maximum a posteriori parameter values for the random probe condition. When assuming across-trial variation, the precision value for each trial was selected at random from one of the three randomly drawn precision values. Error was simulated by sampling from a von Mises distribution with the drawn precision value. For each participant, the resulting error distributions were fit with the variable-precision model, yielding parameter estimates that matched the random probe data (mean 20.2° and s.d. 6.4°; comparable to Fig. 5 , red line). When assuming within-trial variation, we selected the best precision value from the three that were randomly sampled. These values were used to simulate error responses that were then fit with the variable-precision model ( Fig. 5 , blue line, mean 15.4° and s.d. 5.0°). How to cite this article: Fougnie D. et al. Variability in the quality of visual working memory. Nat. Commun. 3:1229 doi: 10.1038/ncomms2237 (2012).